NIR-excitable heterostructured upconversion perovskite nanodots with improved stability There is a great need to develop heterostructured nanocrystals which combine two or more different materials into single nanoparticles with combined advantages. Lead halide perovskite quantum dots (QDs) have attracted much attention due to their excellent optical properties but their biological applications have not been much explored due to their poor stability and short penetration depth of the UV excitation light in tissues. Combining perovskite QDs with upconversion nanoparticles (UCNP) to form hybrid nanocrystals that are stable, NIR excitable and emission tunable is important, however, this is challenging because hexagonal phase UCNP can not be epitaxially grown on cubic phase perovskite QDs directly or vice versa. In this work, one-pot synthesis of perovskite-UCNP hybrid nanocrystals consisting of cubic phase perovskite QDs and hexagonal phase UCNP is reported, to form a watermelon-like heterostructure using cubic phase UCNP as an intermediate transition phase. The nanocrystals are NIR-excitable with much improved stability. There is increasing interest in developing heterostructured nanocrystals that combine two or more different materials into single nanoparticles with combined advantages. For example, heterostructured quantum dots (QDs) such as InP/ZnS, CdSe/CdS/ZnS, Si/CdS, PbSe/PbS, and CdSe/CdTe QDs have been synthesized and have exhibited significantly improved optical and electrical properties as compared to their individual constituents [1] , [2] . QDs are semiconductor nanoparticles whose excitons are limited to the Bohr radius in three-dimensional space, showing the quantum confinement effect [3] . Traditional quantum dots are made of compounds of the IV, II−VI, IV−VI, III−V, and I−III−VI groups, such as Si, CdTe, CdSe, ZnO, PbS, InP, CuInS 2 QDs, etc [4] , [5] . In recent years, lead halide perovskite QDs have attracted much attention due to their excellent optical properties such as high photoluminescence quantum yield (PLQY) up to 100% [6] , [7] , [8] , large UV absorption cross section [9] , tunable emission over the entire visible spectrum [10] , [11] , long carrier diffusion length, and high carrier mobility [12] , which make them suitable for use in high-performance solar cells, light-emitting diodes (LEDs), lasers, and photodetectors [10] , [11] , [12] , [13] , [14] . However, perovskites have poor stability which limits their applications. Furthermore, their use in biological and medical applications is also very limited due to the low penetration depth of UV light in biological tissues. As compared to perovskite QDs, lanthanide-doped upconversion nanocrystals (UCNP) such as NaYF 4 :Yb,Tm have good stability and much higher multi-photon absorption efficiency under NIR excitation using low-cost continuous-wave (CW) lasers [15] , [16] . UCNP have been used in deep tissue fluorescence imaging and phototherapy due to deep penetration of NIR light in biological tissues [17] , [18] , [19] , [20] . However, UCNP have fluorescence emissions at fixed wavelengths only and their emission colors are not tunable and as such their use in multiplexed bioimaging or bioassays is limited. Combining perovskite QDs with UCNP to form hybrid nanocrystals with a heterostructure that are stable, NIR excitable and emission tunable may address the above-mentioned issues. Some studies have been performed to synthesize hybrid perovskite nanocrystals with semiconductor quantum dots with small crystal phase-mismatch such as CsPbBr 3 -CdS [21] , CsPbI 3 -PbS [22] , and CsPbBr 3 -TiO 2 [23] and bulk materials, such as MAPbI 3 -PbS [24] and CsPbX 3 -PbS (X = Cl, Br, and I) [25] . Previous attempts have been made to synthesize UCNP-perovskite nanohybrids. The synthesis of NaYF 4 :Yb,Tm@CH 3 NH 3 PbBr 3 nanohybrids via an innovative strategy consisting of using cucurbituril to anchor the perovskite nanoparticles firmly and closely to the upconversion nanoparticles has been previously achieved [26] . This is a typical A + B synthesis strategy. Material A and B were first synthesized, and an intermediate molecule cucurbituril was used to link the two materials to obtain AB composite material. The composite of perovskite NWs and UCNPs was synthesized at room temperature using PVP as a template [27] . First, the PVP-modified UCNPs were synthesized, and they were mixed with Pb(OA) 2 , which was a perovskite NWs precursor. l-cysteine was added and dispersed in isopropanol solution, and CH 3 NH 3 Br, another precursor of NWs, was added to obtain an AB composite. It is typical to synthesize material A first and then rely on the template method to get the composite material of AB during the synthesis process of material B. They all rely on the action of chemical bonds to connect the two synthetic materials, while we have creatively introduced the intermediate synthesis of crystal phase by controlling the crystal growth, and use the phase-transition characteristics to obtain heterojunction materials with excellent optical properties. However, it remains a challenge to synthesize perovskite/UCNP heterostructured nanocrystals due to the structural difference between cubic-phase perovskite QDs and hexagonal-phase UCNP and lack of a good understanding of the growth/formation mechanism. Going beyond perovskites and UCNP, this has posed a challenge in synthesizing heterostructured nanocrystals consisting of two or more different crystal phases with structural and lattice mismatch and a generic strategy must be developed. In general, some stringent requirements must be met for making heterostructured nanocrystals: (I) crystal structure matching. Cubic-phase CsPbBr 3 crystals can grow together with cubic-phase CdS or PbS crystals [21] , [25] ; (II) lattice parameter matching. MAPbI 3 –PbS lattice mismatch was as small as 4.9% [24] ; (III) similar reaction temperature and condition [21] . There are two strategies for synthesizing A–B hybrid nanocrystals with two different crystals A and B: (I) monodispersed A nanocrystals are synthesized first and then B is epitaxially grown on the surface of A nanocrystals to form a core-shell structure. (II) A and B are synthesized in the same solution simultaneously to produce hybrid nanocrystals with A embedded in B or B embedded in A. Both strategies require A and B to have the same crystal structure and closely matched structural and lattice parameters. For synthesizing perovskite–UCNP hybrid nanocrystals, in this work CsPbBr 3 -NaYF 4 :Yb,Tm, strategy II is adopted. Multiple CsPbBr 3 perovskite QDs are embedded in the NaYF 4 :Yb,Tm UCNP to ensure there is sufficient absorption of NIR excitation light and efficient energy transfer from the UCNP to perovskite QDs. On the other side, it has been widely reported that CsPbBr 3 perovskite QDs have very poor stability in water [23] , [28] . Embedding them in the UCNP will help prevent them from dissolving in water. The challenge to overcome is how to embed cubic-phase CsPbBr 3 QDs in hexagonal-phase NaYF 4 :Yb,Tm UCNP to form hybrid nanocrystals in the same synthetic solution by one-pot synthesis. It is noted that the lattice mismatch between cubic-phase CsPbBr 3 QDs and NaYF 4 :Yb,Tm UCNP is small, 5.9% only. Our hypothesis is those hybrid nanocrystals consisting of cubic-phase CsPbBr 3 QDs and cubic-phase NaYF 4 :Yb,Tm UCNP can be first prepared in one-pot based on co-precipitation method due to small crystal structure mismatch and similarity in synthetic conditions. Phase transition of the UCNP from cubic phase to hexagonal phase is then induced by heating to a higher temperature, resulting in the formation of hybrid nanocrystals with cubic phase CsPbBr 3 QDs embedded in hexagonal-phase NaYF 4 :Yb,Tm UCNP [29] . In this work, we have demonstrated the successful synthesis of monodispersed and oval-shaped watermelon-like hybrid nanocrystals consisting of small cubic-phase CsPbBr 3 QDs (watermelon seeds) embedded in hexagonal-phase NaYF 4 :Yb,Tm UCNP (watermelon pulp) with a thin NaYF 4 :Yb,Tm shell (watermelon skin). The hybrid nanocrystals emit characteristic green fluorescence of the CsPbBr 3 QDs upon UV excitation and UV-blue fluorescence of the NaYF 4 :Yb,Tm UCNP upon NIR excitation, demonstrating the co-existence of both CsPbBr 3 phase and NaYF 4 :Yb,Tm phase in the same structure, and green fluorescence upon NIR excitation when the NaYF 4 :Yb,Tm phase absorbs NIR light and transfers the energy to the CsPbBr 3 phase. This has opened a new way of synthesizing heterostructured nanocrystals with two distinctly different crystal phases via an intermediate transition phase and the strategy could be applied to many other materials. Synthesis of CsPbBr 3 QDs and NaYF 4 :Yb,Tm UCNP CsPbBr 3 QDs with regular cubic shape were first synthesized based on Kovalenko’s method [30] . The size of the CsPbBr 3 QDs was 12.6 nm, and the diffraction peaks at 2 θ = 15.2, 21.6, 26.5 30.6, 34.4, 37.8, 43.9, 46.7, 49.4, 54.5, and 59.3° correspond to diffractions from the {100}, {110}, {111}, {200}, {210}, {211}, {220}, {300}, {310}, {222}, and {321} planes of the cubic-phase CsPbBr 3 (PDF# 00-054-0752) (Supplementary Figs. 1 and 2 ). To analyze the optical properties, the UV−vis absorption spectra, and the PL emission and excitation spectra (Supplementary Fig. 3 ) was obtained from the colloidal solution of the CsPbBr 3 nanocrystals. The PL emission spectrum showed a peak position at 515 nm and showed a strong green fluorescence under 365 nm excitation (Supplementary Fig. 3A ). The absorption onset of CsPbBr 3 nanocrystals was around 510 nm (Supplementary Fig. 3B ). The time-resolved PL decay of CsPbBr 3 showed average PL decay lifetimes was 18.4 ns (Supplementary Fig. 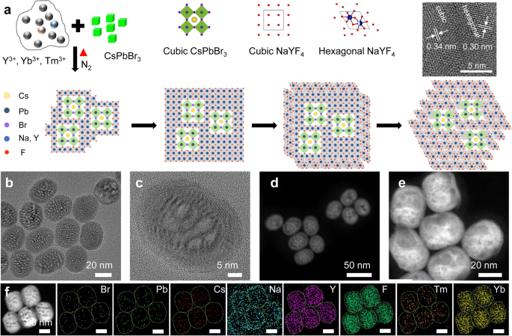Fig. 1: Synthesis of CsPbBr3-NaYF4:Yb,Tm hybrid nanocrystals. aSchematic showing the formation of heterostructured CsPbBr3–NaYF4: Yb,Tm nanocrystals,b,cTEM andd,eSTEM images of heterostructured CsPbBr3–NaYF4:Yb,Tm nanocrystals.fElemental mapping of heterostructured CsPbBr3–NaYF4:Yb,Tm nanocrystals. Scale bars inf, 20 nm. 3C and Supplementary Table 1 ). NaYF 4 :30%Yb,0.5%Tm nanocrystals were synthesized by the high-temperature co-precipitation method [31] . When the temperature reached 300 °C, NaYF 4 :30%Yb and 0.5%Tm nanocrystals with a size of about 5 nm were synthesized, and they emitted a weak fluorescence under 980 nm excitation (Supplementary Fig. 5 ). At 300 °C for 60 min, uniform NaYF 4 :30%Yb,0.5%Tm nanocrystals with a size of 32.5 nm were synthesized, and they emitted a strong blue fluorescence under 980 nm excitation (Supplementary Fig. 6 ). According to the XRD results (Supplementary Fig. 7 ), the diffraction peaks at 2 θ = 17.2, 30.1, 30.8, 34.6, 39.6, 43.5, 46.5, 52.1, 53.1, 53.7, and 55.2° correspond to diffractions from the {100}, {110}, {101}, {200}, {111}, {201}, {210}, {002}, {300}, {211}, and {102} planes of the hexagonal-phase NaYF 4 (JCPDS: 00-016-0334). Synthesis of heterostructured nanocrystals As shown in Fig. 1a , cubic-phase NaYF 4 :Yb,Tm UCNP can be epitaxially grown on the surface of cubic-phase CsPbBr 3 QDs due to the similarity in the crystal structure and lattice. When the temperature is increased, UCNP is converted from cubic to hexagonal phase, while cubic-phase CsPbBr 3 QDs remain unchanged so hexagonal-phase UCNP is formed on the surface of cubic-phase CsPbBr 3 QDs. CsPbBr 3 -NaYF 4 :Yb,Tm hybrid nanocrystals were synthesized using a high-temperature co-precipitation method. Their formation and crystal structures were studied. CsPbBr 3 QDs with regular cubic shape were first synthesized based on Kovalenko’s method (Supplementary Fig. 1 ) [11] , and then added to the precursor solution for UCNP synthesis which consists of various lanthanide ions such as Y 3+ , Yb 3+ , and Tm 3+ and surfactants, such as oleic acid (OA) and octadecylene (ODE). As shown in Fig. 1b–e , heterostructured nanocrystals were formed with the CsPbBr 3 QDs embedded in the NaYF 4 :Yb,Tm UCNP, to form a structure similar to that of watermelon with multiple seeds. The average size of the nanocrystals was ~37 nm, and the outer shell was ~3.7-nm thick (Fig. 1c ). CsPbBr 3 QDs were found to be in the middle region of the nanocrystals with distinct crystal boundary formed between the CsPbBr 3 QDs and UCNP from the bright- and dark-field TEM images. The heterostructure interface can be clearly seen from the HRTEM diagram (Supplementary Fig. 8 ), and the area segmented by the arc presents obvious light and dark patterns. Above the arc is the cubic-phase CsPbBr 3 crystals and below the arc is the hexagonal-phase NaYF 4 :Yb,Tm crystals. The cubic-phase NaYF 4 :Yb,Tm is a metastable crystalline phase, which led to the formation of irregular small cubic-phase CsPbBr 3 crystals within the heterogeneous junction, thus making the interface of heterogeneous junction irregular. From HRTEM, STEM, and elemental imaging results (Supplementary Fig. 9 ), it can be clearly seen that the perovskites in the heterostructured nanocrystals were small irregular particles with a size of 6–12 nm. At 250 °C, the heterostructured nanocrystals were composed of a cubic-phase UCNPs and cubic-phase perovskites. The cubic-phase UCNPs has a high-temperature metastable crystalline phase, which led to the irregular growth of perovskites in the heterojunction. Subsequently, under the effects of thermodynamics (250–300 °C), the cubic-phase UCNP transited to the hexagonal phase. At this time, the epitaxial growth was mainly due to the hexagonal-phase UCNP, and most of the perovskite stopped growing due to the mismatch of crystal phases. As shown in Fig. 1f , eight elements including Br, Pb, Cs, Na, Y, F, Tm, and Yb were distributed in the nanocrystal structure (Supplementary Fig. 10 ). The elemental mapping images showed that Na, Y, F, Tm, and Yb ions which constitute the NaYF 4 :Yb,Tm UCNP were uniformly distributed throughout the hybrid nanocrystals, while Br, Pb, and Cs ions which make up CsPbBr 3 QDs were located in the middle part. This could also be seen from the images of single-particle element imaging (Supplementary Fig. 11 ), supporting that the hybrid nanocrystals were formed with the CsPbBr 3 QDs embedded in the NaYF 4 :Yb,Tm UCNP. According to the XPS results, the concentration ratio of CsPbBr 3 and NaYF 4 :Yb,Tm in the heterostructured nanocrystals was 1:59. 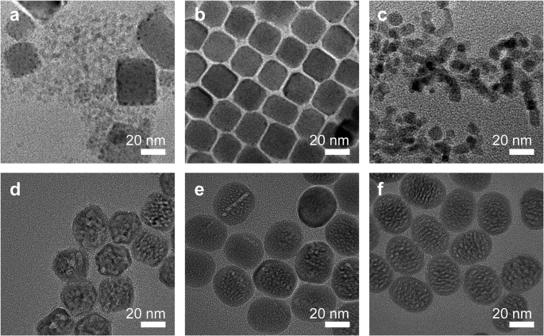Fig. 2: Nanocrystal heterostructure formation during heat treatment. TEM images of heterostructured CsPbBr3–NaYF4: Yb,Tm nanocrystals collected during the synthesis at different temperatures.a150 °C,b200 °C,c250 °C,d300 °C—0 min,e300 °C-30 min,f300 °C—60 min. (Supplementary Table 2 ). Fig. 1: Synthesis of CsPbBr 3 -NaYF 4 :Yb,Tm hybrid nanocrystals. a Schematic showing the formation of heterostructured CsPbBr 3 –NaYF 4 : Yb,Tm nanocrystals, b , c TEM and d , e STEM images of heterostructured CsPbBr 3 –NaYF 4 :Yb,Tm nanocrystals. f Elemental mapping of heterostructured CsPbBr 3 –NaYF 4 :Yb,Tm nanocrystals. Scale bars in f , 20 nm. Full size image Nanocrystal heterostructure formation during heat treatment The formation of the CsPbBr 3 -NaYF 4 :Yb,Tm hybrid nanocrystals was studied by TEM measurement of the samples collected at different temperatures during the heat-treatment process. From the literature, it was reported that cubic-phase CsPbBr 3 crystals (5.83 Å) and cubic-phase NaYF 4 crystals (5.47 Å) have a small lattice mismatch of ~5.9%, suggesting that theoretically it is possible to grow cubic phase CsPbBr 3 crystals on cubic-phase NaYF 4 crystals epitaxially or vice versa [32] , [33] , [34] . In this study, pre-made cubic-phase CsPbBr 3 QDs were added to the precursor solution to synthesize NaYF 4 :Yb,Tm UCNP, so it is a high probability that NaYF 4 :Yb,Tm crystals were grown on the surface of CsPbBr 3 QDs, evidenced from the dark spots formed on the surface of the cubic-shape nanocrystals at 150 °C and 200 °C, as shown in Fig. 2a, b . This is similar to cubic-phase CsPbX 3 –PbS hybrid nanocrystals formed under a similar condition [25] . The temperature was subsequently increased to 250 °C, resulting in much smaller nanocrystals with a size of ~12 nm (Fig. 2c ). Besides poor chemical stability in water, poor thermostability of CsPbBr 3 QDs has also been well reported [35] , [36] . High temperature may cause the oxidation and hydration and eventually the decomposition of CsPbBr 3 QDs. At 250 °C, the size of the nanocrystals was apparently much smaller as compared to a lower temperature, suggesting that CsPbBr 3 QDs started to decompose partially. This is usually considered a problem for perovskite QDs; however, in this study, the smaller size of perovskite QDs caused by partial decomposition makes it possible to synthesize small perovskite–UCNP hybrid nanocrystals. On the other side, the cubic phase is dominant in the NaYF 4 nanocrystals formed at 250 °C, as previously reported [29] , [37] , [38] . The small hybrid nanocrystals served as the seeds for further growth of the NaYF 4 :Yb,Tm UCNP. The average size of the nanocrystals increased to 30.6 nm when the temperature reached 300 °C (Fig. 2d ). With the extension of the insulation time to 30 and 60 min, the size continued to increase to 34.5 nm and 37.1 nm, respectively (Fig. 2e, f ). Their morphology changed from square or hexagonal to ellipsoidal shape. In addition, multiple cores were clearly observed in the middle region of the perovskite–UCNP hybrid nanocrystals during the thermal insulation process (Supplementary Fig. 12 ), which was consistent with the previous elemental mapping results. Fig. 2: Nanocrystal heterostructure formation during heat treatment. TEM images of heterostructured CsPbBr 3 –NaYF 4 : Yb,Tm nanocrystals collected during the synthesis at different temperatures. a 150 °C, b 200 °C, c 250 °C, d 300 °C—0 min, e 300 °C-30 min, f 300 °C—60 min. Full size image Luminescence emission profile The fluorescence emission of nanocrystals is dependent on the crystal structure and phases. Fluorescence emission spectra of the perovskite–UCNP hybrid nanocrystals collected at different temperatures were measured under excitation at 980 nm and 365 nm, respectively, and used to study the crystal phase formation and transition during the synthesis of the hybrid nanocrystals. As shown in Fig. 3a , the hybrid nanocrystals had three different states of luminescence: it emitted blue and cyan fluorescence under 980 nm excitation and green fluorescence under 365 nm excitation. When the temperature was increased from 150 °C to 250 °C, upconversion luminescence was weak and there was no characteristic green fluorescence emission of CsPbBr 3 QDs at 515 nm under 980 nm excitation, indicating that there is no energy transfer from the NaYF 4 :Yb,Tm UCNP to CsPbBr 3 QDs due to the low luminescence efficiency of cubic-phase NaYF 4 :Yb,Tm UCNP formed at low temperature [38] , [39] . The intensity of the green fluorescence of CsPbBr 3 QDs under 365 nm excitation decreased due to the partial decomposition of the QDs. When the temperature was further increased to 300 °C, the hybrid nanocrystals exhibited UV/blue upconversion fluorescence under 980 nm excitation (Fig. 3b ), with emission peaks located at 292 nm ( 1 I 6 → 3 F 4 ), 347 nm ( 1 I 6 → 3 F 4 ), 362 nm ( 1 D 2 → 3 H 6 ), 450 nm ( 1 D 2 → 3 F 4 ), and 478 nm ( 1 G 4 → 3 H 6 ), and green fluorescence at 522 nm corresponding to the emission of CsPbBr 3 QDs, suggesting a significant energy transfer from the NaYF 4 :Yb,Tm UCNP to CsPbBr 3 QDs and formation of hexagonal-phase NaYF 4 :Yb,Tm UCNP. It has been reported that hexagonal-phase NaYF 4 :Yb,Tm UCNP emits much stronger upconversion fluorescence as compared to its cubic phase [38] , [39] , [40] . During the process of maintaining the temperature at 300 °C for 0 to 60 min, the intensity of the green fluorescence emission peak increased, suggesting an increased energy transfer from the NaYF 4 :Yb,Tm UCNP to CsPbBr 3 QDs. Meanwhile, at 300 °C, the hybrid nanocrystals emitted strong green fluorescence at 525 nm under 365 nm excitation which was corresponding to CsPbBr 3 QDs (Fig. 3c ). The absorption of the heterostructure composite of CsPbBr 3 –NaYF 4 :Yb,Tm nanocrystals were around 510 nm. The excitation spectrum showed that the heterostructure composite of CsPbBr 3 –NaYF 4 :Yb,Tm nanocrystals exhibited the strongest peak at 475 nm monitored at the emission wavelength of 525 nm, which is in good agreement with the result from the UV–vis absorption spectrum (Supplementary Fig. 13 ). During the process of nanocrystals formation and growth, the heterostructured nanocrystal at 250 °C was composed of cubic-phase UCNPs and cubic-phase CsPbBr 3 . When the temperature increased to 300 °C and incubated for 60 min, the cubic-phase UCNPs changes to the hexagonal phase and resulted in the heterostructured nanocrystals of the hexagonal-phase UCNPs and cubic-phase CsPbBr 3 formation. 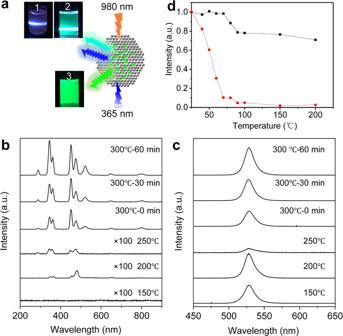Fig. 3: Fluorescence of CsPbBr3–NaYF4:Yb,Tm hybrid nanocrystals. aPhotographs showing different color fluorescence emitted from the heterostructured CsPbBr3-NaYF4:Yb,Tm nanocrystals collected during the synthesis under different conditions (state 1, 300 °C—0 min, state 2, 300 °C—60 min, both under 980 nm excitation, state 3, 300 °C—60 min, under 365 nm excitation).b,cFluorescence emission spectra of heterostructured CsPbBr3–NaYF4:Yb,Tm nanocrystals at different temperatures under 980 nm and 365 nm excitations, respectively.dFluorescence intensity of CsPbBr3nanocrystals (red) and heterostructured CsPbBr3–NaYF4:Yb,Tm nanocrystals (black) collected at different temperatures under 365 nm excitation. The PLQY of these heterostructured nanocrystals under excitation at 980 nm were as follows: 150 °C (0%), 200 °C (0%), 250 °C (0.02%), 300 °C—0 min (0.15%), and 300 °C—60 min (0.25%) (Supplementary Table 3 ). Similarly, the PLQY of these heterostructured nanocrystals increased from 0.02% to 0.139% under the 980 nm excitation. This PLQY increase was a result of the NaYF 4 phase transition from cubic to hexagonal. The hexagonal-phase NaYF 4 has a much higher fluorescence efficiency as compared to its cubic phase. The PLQY of these heterostructured nanocrystals under 365 nm excitation were as follows: 150 °C (53%), 200 °C (35%), 250 °C (12%), 300 °C—0 min (23%), and 300 °C—60 min (21%) (Supplementary Table 3 ). Under the excitation of 365 nm, the peak position of heterostructured nanocrystals was 525 nm. The PLQY increased from 12% to 23% during the heterostructured nanocrystal phase-transition process. 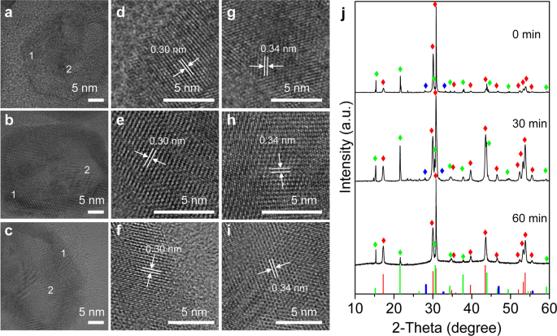Fig. 4: Structural analysis of CsPbBr3-NaYF4:Yb,Tm hybrid nanocrystals. HRTEM images of heterostructured CsPbBr3-NaYF4:Yb,Tm nanocrystals collected during the synthesis after heated at 300 °C for different time:a0 min,b30 min,c60 min.d–fEnlarged images of region 1 ina,b, andc, respectively.g–iEnlarged images of region 2 ina,b, andc, respectively.jX-ray diffraction (XRD) patterns of the three samples. Hexagonal NaYF4, red color (JCPDF#00-016-0334), cubic NaYF4, blue color (JCPDF #01-077-2042), cubic CsPbBr3, green color (JCPDF #00-054-0752). The fluorescence quantum efficiency of the conventional CsPbBr 3 nanocrystals was 65%, and fluorescence quenching occurred after CsPbBr 3 nanocrystals was kept at 300 °C for 60 min (Supplementary Table 3 and Supplementary Table 4 ). On the other hand, the PLQY of the perovskite within the heterostructured nanocrystals excited by 365 nm was about 21% after being kept at 300 °C for 60 min far higher than that of the conventional CsPbBr 3 nanocrystals at 300 °C for 60 min (Supplementary Table 4 ). The conventional CsPbBr 3 nanocrystals were kept at 300 °C for 60 min, resulting in very small-sized particles and very weak fluorescence (Supplementary Fig. 4 ). This is because the conventional CsPbBr 3 nanocrystals shrank in size, dissolved, and their crystal structure was destroyed at 300 °C after 60 min. The heterojunctured nanocrystals have strong fluorescence at the 525 nm peak under 365 nm excitation, which fully indicated that the cubic-phase and hexagonal-phase UCNP have an obvious protective effect on CsPbBr 3 nanocrystals at high temperature. The hybrid nanocrystals were reheated reheated to different temperatures of 25 °C, 40 °C, 50 °C, 60 °C, 70 °C, 80 °C, 90 °C, 100 °C, 150 °C, and 200 °C, and compared to pure CsPbBr 3 perovskite QDs. When the temperature was increased to 200 °C, the intensity of CsPbBr 3 QDs quickly reduced to 2% while the intensity of the hybrid nanocrystals dropped to 71% only, showing the protection of the CsPbBr 3 QDs by the UCNP at high temperature (Fig. 3d and Supplementary Fig. 14 ). Relative fluorescence intensity of the heterostructured CsPbBr 3 –NaYF 4 :Yb,Tm hybrid nanocrystals still maintained around 90% during the heating process under 980 nm excitation (Supplementary Fig. 15 ). The hybrid nanocrystals maintained the luminescent properties of both perovskite QDs and UCNP and improved the stability of perovskite QDs at high temperatures. Fig. 3: Fluorescence of CsPbBr 3 –NaYF 4 :Yb,Tm hybrid nanocrystals. a Photographs showing different color fluorescence emitted from the heterostructured CsPbBr 3 -NaYF 4 :Yb,Tm nanocrystals collected during the synthesis under different conditions (state 1, 300 °C—0 min, state 2, 300 °C—60 min, both under 980 nm excitation, state 3, 300 °C—60 min, under 365 nm excitation). b , c Fluorescence emission spectra of heterostructured CsPbBr 3 –NaYF 4 :Yb,Tm nanocrystals at different temperatures under 980 nm and 365 nm excitations, respectively. d Fluorescence intensity of CsPbBr 3 nanocrystals (red) and heterostructured CsPbBr 3 –NaYF 4 :Yb,Tm nanocrystals (black) collected at different temperatures under 365 nm excitation. Full size image Exploration of the energy-transfer mechanism The Förster resonance energy transfer (FRET) and the emission reabsorption (ERA) were the two main energy-transfer processes. The changes in fluorescence lifetime are directly associated with FRET, but not with ERA. Efficient FRET between NaYF 4 :Yb,Tm donors and CsPbBr 3 acceptors will only take place at short distances. Indeed, the fluorescence average lifetime reduction of the blue emission at 478 nm from 0.66 ms of the NaYF 4 :30%Yb,0.5%Tm nanocrystals to 0.29 ms of the CsPbBr 3 –NaYF 4 :Yb,Tm nanocrystals (Supplementary Fig. 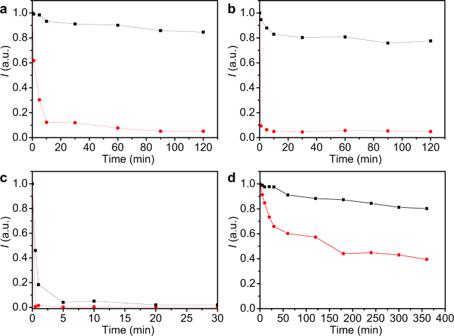Fig. 5: Stability analysis of CsPbBr3–NaYF4:Yb,Tm hybrid nanocrystals. PL intensity test was used to monitor the stabilities of CsPbBr3(red) and the heterostructure composite of CsPbBr3–NaYF4:Yb,Tm nanocrystals (black) in cyclohexane and ethanol (v/v = 9: 1) mixed solvent (a), cyclohexane and ethanol (v/v = 1: 1) mixed solvent (b), water solvent (c), and continuous ultraviolet light irradiation (d) under 365 nm excitation. 16 and Supplementary Table 5 ) suggested that the energy transfer from NaYF 4 :Yb,Tm to CsPbBr 3 in the heterostructure follows a typical FRET process [27] , [41] . The FRET efficiency can be calculated with the equation Eff = 1 − τ D–A /τ D , where Eff is the energy transfer efficiency, τ D–A is the effective lifetime of a donor conjugated with an acceptor, and τ D is the effective lifetime of a donor in the absence of an acceptor. The FRET efficiency of the CsPbBr 3 –NaYF 4 :Yb,Tm nanocrystals calculated was 56%, which justifies our design for an efficient energy transport strategy. The fluorescence lifetime of the mixed CsPbBr 3 and NaYF 4 :Yb,Tm is 0.59 ms, which only reduces 0.07 ms compared with the NaYF 4 :30%Yb,0.5%Tm NPs fluorescence lifetime of 0.66 ms, and the efficiency of FRET is calculated to be 11%, far lower than the energy transfer efficiency of FRET in the heterogeneous junction (Supplementary Figs. 16 , 17 and Supplementary Tables 5 , 6 ). Therefore, the energy transfer process of the mixed CsPbBr 3 and NaYF 4 :Yb,Tm is mainly EAU, which is different from that of FRET in heterostructured CsPbBr 3 -NaYF 4 :Yb,Tm hybrid nanocrystals. In addition, the fluorescence lifetime of the perovskites has increased from 18 ns to 0.37 ms (Supplementary Fig. 18 and Supplementary Table 7 ). By changing the number of perovskites, we have changed the ratio between the perovskite and UCNP in the heterostructured nanocrystals, and obtained 0.2-fold and fivefold CsPbBr 3 –NaYF 4 :Yb,Tm nanocrystals. The fluorescence lifetime of the onefold heterostructured nanocrystal is 0.29 ms (Supplementary Fig. 19 and Supplementary Table 8 ). The fluorescence lifetime of the 0.2-fold heterostructured nanocrystal increased to 0.49 ms, while that of the fivefold heterostructured nanocrystal decreased to 0.25 ms (Supplementary Table 8 ). As compared to the FRET efficiency of the onefold heterostructured nanocrystal, 56%, the FRET efficiency of the 0.2-fold heterostructured nanocrystal was reduced to 25.8%. On the other hand, the FRET efficiency of the fivefold heterostructured nanocrystal increased to 62.1% (Supplementary Table 9 ). Therefore, it shows that the decrease in the perovskite/UCNP ratio resulted in increased fluorescence lifetime and decreased FRET efficiency. Compared to the fluorescence spectra of pure UCNP under 980 nm excitation, the absorption of the fluorescence emitted from UCNP increases with the increase of the perovskite amount (Supplementary Fig. 20 ). Regulation of optical properties The heterojunction nanocrystals synthesized by us could undergo anion exchange with Cl − and I − to control the energy transfer and luminescence performance. Under the 980 nm excitation, the 525 nm fluorescence peak emitted by the perovskites within the heterogeneous crystals was shifted to 578 nm after the addition of I − . On the other hand, this same peak was shifted to 478 nm after the addition of Cl − (Supplementary Fig. 21A ). During the anion exchange in CsPbBr 3 nanocrystals with the introduction of I − into the heterogeneous crystal, and the fluorescence lifetime of CsPbBr 3 nanocrystals in the heterojunction became longer. However, the introduction of Cl − into the heterojunction shortened the fluorescence lifetime of CsPbBr 3 nanocrystals in the heterogeneous crystal [42] , thus affecting the energy transfer efficiency. Under the 365 nm excitation, the 525 nm fluorescence peak emitted from the heterogeneous crystal was blue shifted to 479 nm and red shifted to 578 nm, respectively (Supplementary Fig. 21B ). Therefore, this heterojunction nanocrystal structure was able to regulate the energy-transfer process and optical properties from NaYF 4 :Yb,Tm to CsPbBr 3 nanocrystals via anion exchange. Compared with pure UCNPs, heterogeneous crystals can not only regulate their optical properties through anion exchange but also change the composition of CsPbX 3 nanocrystals in heterogeneous crystals. With the ratios of perovskites to UCNPs kept unchanged and only the perovskite composition was changed, we have obtained the heterostructured CsPbBr 2 /Cl 1 -NaYF 4 :Yb,Tm nanocrystals and the heterostructured CsPbBr 2 /I 1 -NaYF 4 :Yb,Tm nanocrystals. The size of the heterostructured CsPbBr 2 /Cl 1 -NaYF 4 :Yb,Tm and CsPbBr 2 /I 1 -NaYF 4 :Yb,Tm nanocrystals were 42.3 nm and 39.6 nm, respectively (Supplementary Fig. 24A, B ). The irregular small particles of perovskite in the heterostructured nanocrystals were also observed. According to the fluorescence spectrum under the excitation of 980 nm (Supplementary Fig. 24C, D ), the emission peak of the perovskites in the heterostructured CsPbBr 2 /Cl 1 -NaYF 4 :Yb,Tm nanocrystals was shifted left to 477 nm, while the emission peak of the perovskites in the heterostructured CsPbBr 2 /I 1 -NaYF 4 :Yb,Tm nanocrystals was shifted right to 542 nm. Under 365 nm excitation, the fluorescence peaks of the heterostructured CsPbBr 2 /Cl 1 -NaYF 4 :Yb,Tm and CsPbBr 2 /I 1 -NaYF 4 :Yb,Tm nanocrystals were 478 nm and 542 nm (Supplementary Fig. 24E, F ), respectively. These peaks matched with the upconversion fluorescence peaks of CsPbX 3 in the heterostructured nanocrystals which indicated that the NaYF 4 :Yb,Tm has a protective effect on the structure of perovskite at high temperature. The fluorescence lifetimes of the heterostructured CsPbBr 2 /Cl 1 -NaYF 4 :Yb,Tm and CsPbBr 2 /I 1 -NaYF 4 :Yb,Tm nanocrystals at the 478 nm peak were 0.23 ms and 0.48 ms, respectively (Supplementary Fig. 24G-H and Supplementary Table 10 ). Therefore, we have shown that our synthesis strategy is compatible to synthesize heterogeneous junctions composed of different types of UCNPs and perovskites. If the aforementioned three conditions were met, different types of heterogeneous junction products such as PbS-UCNPs, CdS-UCNPs can be obtained. Phase transition At 250 °C, the heterojunction nanocrystals mainly contained cubic-phase CsPbBr 3 crystals and cubic-phase NaYF 4 :Yb,Tm crystals according to the standard data of JCPDS# 00-054-0752 and JCPDS# 00-016-0334 (Supplementary Fig. 25 ). The 2 θ of the {100} crystal plane of the cubic-phase CsPbBr 3 crystals has increased from 15.18° to 15.3°, and the lattice spacing has decreased. On the other hand, the 2 θ of the {100} crystal plane of the cubic-phase NaYF 4 :Yb,Tm crystals has decreased from 28.2° to 27.8°, which further indicated that the lattice strain was generated by the heterojunction nanocrystals at 250 °C. In order to understand the phase transition during the process of maintaining the temperature at 300 °C for 0 to 60 min, lattice spacing and XRD measurements for the above samples were performed. In this process, as seen in Fig. 4a–i , the lattice distance on the surface of the hybrid nanocrystals was 0.3 nm in accordance with the {110} lattice spacing of hexagonal-phase NaYF 4 UCNP (JCPDS: 00-016-0334), while the lattice distance in the middle was 0.34 nm corresponding to the {111} lattice spacing of cubic-phase CsPbBr 3 QDs (JCPDS: 00-054-0752). The high-resolution TEM images confirmed that the two crystals were grown together and well combined which is very important to ensure a highly efficient energy transfer between them when excited at 980 nm. At 300 °C, XRD results in Fig. 4j showed that the nanocrystals mainly contained cubic-phase CsPbBr 3 crystals and hexagonal-phase NaYF 4 crystals, according to the standard data of JCPDS# 00-054-0752 and JCPDS# 00-016-0334. Very weak peaks of cubic-phase NaYF 4 crystals (JCPDS: 01-077-2042) were also observed. With the extension of the thermal insulation time, the cubic-phase NaYF 4 crystals transformed to hexagonal-phase NaYF 4 crystals and finally disappeared, resulting in an increase in the relative proportion of hexagonal NaYF 4 crystals (Supplementary Fig. 26 ), so only cubic-phase CsPbBr 3 crystals and hexagonal-phase NaYF 4 crystals co-existed in the hybrid nanocrystals. The process of phase transition led to the formation of crystal boundary in the nanocrystal structure, which was confirmed with HRTEM results. When cubic-phase NaYF 4 crystals transformed to the hexagonal phase with high fluorescence efficiency, upconversion fluorescence was enhanced, which was also consistent with the results of fluorescence measurement. Fig. 4: Structural analysis of CsPbBr 3 -NaYF 4 :Yb,Tm hybrid nanocrystals. HRTEM images of heterostructured CsPbBr 3 -NaYF 4 :Yb,Tm nanocrystals collected during the synthesis after heated at 300 °C for different time: a 0 min, b 30 min, c 60 min. d – f Enlarged images of region 1 in a , b , and c , respectively. g – i Enlarged images of region 2 in a , b , and c , respectively. j X-ray diffraction (XRD) patterns of the three samples. Hexagonal NaYF 4 , red color (JCPDF#00-016-0334), cubic NaYF 4 , blue color (JCPDF #01-077-2042), cubic CsPbBr 3 , green color (JCPDF #00-054-0752). Full size image Stability study The stability in a mixture solution of cyclohexane and ethanol with a ratio of 9:1 or 1:1 has significantly improved as compared to the conventional CsPbBr 3 nanocrystals. We have studied the stability of heterostructure composite of CsPbBr 3 -NaYF 4 :Yb,Tm nanocrystals in a mixture solution of cyclohexane and ethanol with a ratio of 9:1 (Fig. 5a and Supplementary Fig. 27 ) also. The relative fluorescence intensity of the CsPbBr 3 nanocrystals decreased to 12% at 10 min and 5% at 120 min in the mixture solution. On the other hand, the heterostructure composite of CsPbBr 3 -NaYF 4 :Yb,Tm nanocrystals has managed to maintain a relative fluorescence intensity of 93% at 10 min and 85% at 120 min. This result suggests good stability in a mixture of cyclohexane and ethanol with a ratio of 9:1. Furthermore, the relative fluorescence intensity of the CsPbBr 3 nanocrystals quickly decreased to 10% at 1 min and 5% at 120 min in a mixture of cyclohexane and ethanol with a ratio of 1:1 (Fig. 5b and Supplementary Fig. 27 ), whereas the heterostructure composite of CsPbBr 3 -NaYF 4 :Yb,Tm nanocrystals has maintained a relative fluorescence intensity of 95% at 1 min and slowly decrease to 80% after 2 h. This result suggests excellent fluorescence stability in a mixture of cyclohexane and ethanol with a ratio of 1:1. The stability of the heterostructure composite of CsPbBr 3 –NaYF 4 :Yb,Tm nanocrystals in water was still less than ideal. As shown in Fig. 5c , the relative fluorescence intensity of CsPbBr 3 nanocrystals in water solution has decreased to <1% after 30 s, while the relative fluorescence intensity of the heterostructure composite of CsPbBr 3 -NaYF 4 :Yb,Tm nanocrystals was able to remain at 46% in water solution (Supplementary Fig. 28 ). Even though the relative fluorescence intensity decreased to about 4% in 5 min eventually, the stability of these heterostructured nanocrystals in the water has shown slight improvement as compared to the conventional CsPbBr 3 nanocrystals. From the results of solvent stability experiments, it can be inferred that there were bare perovskite crystals on the heterogeneous crystal surface that were not completely covered by NaYF 4 :Yb,Tm nanocrystals. Upon contact with the water molecules, the water molecules infiltrated into the heterogeneous crystal structure along with the perovskite found on the crystal surface. Thus, the perovskite crystal structure in the heterogeneous junction was destroyed and reduced the fluorescence significantly. In addition, we have studied light stability. Under continuous ultraviolet light, the CsPbBr 3 nanocrystals only have a 40% relative fluorescence intensity after 360 min, while heterostructure composite of CsPbBr 3 –NaYF 4 :Yb,Tm nanocrystals maintained an 80% fluorescence intensity (Fig. 5d and Supplementary Fig. 29 ). This result suggests that the heterostructured nanocrystals have good light stability. Fig. 5: Stability analysis of CsPbBr 3 –NaYF 4 :Yb,Tm hybrid nanocrystals. PL intensity test was used to monitor the stabilities of CsPbBr 3 (red) and the heterostructure composite of CsPbBr 3 –NaYF 4 :Yb,Tm nanocrystals (black) in cyclohexane and ethanol (v/v = 9: 1) mixed solvent ( a ), cyclohexane and ethanol (v/v = 1: 1) mixed solvent ( b ), water solvent ( c ), and continuous ultraviolet light irradiation ( d ) under 365 nm excitation. Full size image In summary, heterostructured CsPbBr 3 –NaYF 4 :Yb,Tm nanocrystals were synthesized in one-pot with cubic-phase CsPbBr 3 QDs embedded in hexagonal-phase NaYF 4 :Yb,Tm UCNP to form a structure of watermelon with multiple seeds, using cubic-phase NaYF 4 :Yb,Tm UCNP as an intermediate transition phase. Different phase crystals can not grow on each other epitaxially to form a heterostructure due to unmatched crystal structure and lattice. Synthesizing heterostructured nanocrystals with two or more different crystal phases remains a challenge. We have successfully demonstrated that cubic-phase perovskite QDs and hexagonal-phase UCNP could be combined into a single nanocrystal by introducing an intermediate transition phase into the synthesis. Cubic-phase UCNP was grown on cubic-phase perovskite QDs to form single nanocrystals, followed by a phase transition from cubic-phase UCNP to hexagonal-phase UCNP by heating to a higher temperature, to obtain monodispersed and heterostructured perovskite–UCNP nanocrystals with multiple cubic-phase perovskite QDs embedded in hexagonal-phase UCNP. Going beyond this, a generic strategy has been developed to synthesize heterostructured nanocrystals with different phases based on phase transition and this could be readily applied to many other materials. Chemicals and materials Cesium carbonate (Cs 2 CO 3 , 99.9%), lead bromide (PbBr 2 , 99.9%), lead chloride (PbCl 2 , 99.9%), lead iodide (PbI 2 , 99.9%), yttrium acetate ((CH 3 CO 2 ) 3 Y·xH 2 O, 99.9%), ytterbium acetate ((CH 3 CO 2 ) 3 Yb·4H 2 O, 99.9%), thulium(III) acetate ((CH 3 CO 2 ) 3 Tm·xH 2 O, 99.9%), sodium hydroxide (NaOH, 99%), ammonium fluoride (NH 4 F, 98%), octadecene (ODE, 95%), oleic acid (OA, 90%), oleylamine (OAm, 98%), oleylamine chloride (OAmCl, 99%), oleylamine iodide (OAmI, 99%), cyclohexane (99.9%), and toluene (99.9%) were purchased from Sigma-Aldrich and used as received without further purification. Synthesis of CsPbBr 3 perovskite nanocrystals Cs-oleate was synthesized by reacting Cs 2 CO 3 (0.2 g) with OA (0.6 mL) in octadecene (7.5 mL) and pre-heated to 120 °C before injection. PbBr 2 (0.188 mmol) and 5 mL of ODE were loaded into a 100 mL 3-neck flask, dried under vacuum at 120 °C for 1 h, and mixed with vacuum-dried OAm (0.5 mL) and OA (0.5 mL) under a N 2 atmosphere. The temperature was raised to 150 °C, and 0.6 mL of Cs-oleate solution was rapidly injected. After 5 s, the reaction mixture was cooled in an ice-water bath. Nanocrystals were precipitated by centrifugation at 12,000 rpm and re-dispersed in 10 mL of cyclohexane. Other samples (CsPbBr 2 Cl 1 and CsPbBr 2 I 1 ) with different ratios of Br/Cl or I = 2/1 were synthesized by the same strategy. The other conditions for synthesis and purification remain the same. Synthesis of heterostructured CsPbBr 3 - NaYF 4 : Yb,Tm nanocrystals First, 0.695 mmol Y(CH 3 CO 2 ) 3 , 0.30 mmol Yb(CH 3 CO 2 ) 3 , and 0.005 mmol Tm(CH 3 CO 2 ) 3 were mixed with 6 mL of oleic acid and 15 mL of octadecene in a 50-mL flask and heated to 150 °C. After cooled down to room temperature, 10 mL of methanol solution (100 mg NaOH and 150 mg NH 4 F) were slowly added into the flask, and the solution was stirred for 10 min. The solution was subsequently heated to remove methanol and degassed at 120 °C for 20 min. In all, 1 mL of CsPbBr 3 solution was hot-injected into the precursor solution and then heated to 300 °C for 1 h under N 2 environment. The product was washed twice with cyclohexane by centrifugation for 10 min and dispersed in 20 mL of cyclohexane for further use. The ratio between CsPbBr 3 and NaYF 4 : Yb,Tm nanocrystals could be adjusted. Synthesis of heterostructured CsPbBr 2 Cl 1 - NaYF 4 : Yb,Tm and heterostructured CsPbBr 2 I 1 - NaYF 4 :Yb,Tm nanocrystals In total, 0.695 mmol (CH 3 CO 2 ) 3 Y, 0.30 mmol (CH 3 CO 2 ) 3 Yb, and 0.005 mmol (CH 3 CO 2 ) 3 Tm were mixed with 6 mL of oleic acid and 15 mL of octadecene in a 50-mL flask and heated to 150 °C. After cooled down to room temperature, 10 mL of methanol solution (100 mg NaOH and 150 mg NH 4 F) was slowly added into the flask, and the solution was stirred for 10 min. The solution was subsequently heated to remove methanol and degassed at 120 °C for 20 min. In all, 1 mL of CsPbBr 2 I 1 or CsPbBr 2 I 1 solution was hot-injected into the precursor solution and then heated to 300 °C for 1 h under N 2 environment. The product was washed twice with cyclohexane by centrifugation for 10 min and dispersed in 20 mL of cyclohexane for further use. Anion exchange of heterostructured CsPbBr 3 - NaYF 4 : Yb,Tm nanocrystals The anion-exchange reactions were performed in a 10-mL glass bottle. The heterostructured CsPbBr 3 - NaYF 4 : Yb,Tm nanocrystals (5 mL, 0.05 mol/L) were used as the precursor. For anion exchange, OAmI or OAmCl (20 mg) was dissolved in cyclohexane (20 mL) as the anion source, and add 850 μL of OAmI or 700 μL of OAmCl solution into the heterostructured nanocrystals solution (5 mL) to achieve anion exchange. Anion exchange could be completed in a time period ranging from tens of seconds to a few minutes. After the reaction, the emission peaks of the solution were detected by a spectrofluorometer. Characterization TEM was performed on an FEI Tecnai G2 F20 electron microscope operating at 200 kV. Low-voltage high-resolution STEM measurement was carried out on a double-aberration-corrected Titan TM cubed G2 60−300 S/TEM equipped with Super-XTM technology. The available point resolution is ~0.1 nm at an operating voltage of 60 kV. XRD was measured with a Bruker AXS D8 X-ray diffractometer equipped with monochromatized Cu Kα radiation ( λ = 1.5418 Å). XPS was performed using an achromatic Al Kα source (1486.6 eV) and a double-pass cylindrical mirror analyzer (ULVACPHI 5000 Versa Probe) (Japan). Heterostructured nanocrystals were dissolved in cyclohexane solution at a concentration of 0.05 mol/L, and the upconversion fluorescence spectrum, down-conversion fluorescence spectrum, absorption spectrum, excitation spectrum, and fluorescence lifetime were tested and characterized. Ultraviolet and visible absorption (UV–vis) spectra were recorded with a Shimadzu UV-3600 plus spectrophotometer equipped with an integrating sphere under ambient conditions. Photoluminescence excitation and emission spectra and fluorescence decays were recorded on a FLS980 spectrometer (Edinburgh) equipped with both continuous xenon (450 W) and pulsed flash lamps. Upconversion fluorescence emission spectra were acquired under 980 nm excitation with a CW diode laser (2 W/cm 2 ). Measurement of absolute up- and down-conversion PLQY of nanocrystals was performed using a standard barium sulfate-coated integrating sphere (Edinburgh). The sample chamber was mounted to a FLS980 spectrophotometer. Lifetime was measured with a customized UV to mid-infrared steady-state and phosphorescence lifetime spectrometer (FSP920-C, Edinburgh) equipped with a digital oscilloscope (TDS3052B, Tektronix) and a tunable mid-band Optical Parametric Oscillator pulsed laser as the excitation source (410–2400 nm, 10 Hz, pulse width ≤5 ns, Vibrant 355II, OPOTEK). Fluorescence decay was measured on a Nikon Ni-U Microfluorescence Lifetime system with a 375 nm picosecond laser and a time-correlated single-photon counting system at room temperature.